Light–matter interaction in a microcavity-controlled graphene transistor Graphene has extraordinary electronic and optical properties and holds great promise for applications in photonics and optoelectronics. Demonstrations including high-speed photodetectors, optical modulators, plasmonic devices, and ultrafast lasers have now been reported. More advanced device concepts would involve photonic elements such as cavities to control light–matter interaction in graphene. Here we report the first monolithic integration of a graphene transistor and a planar, optical microcavity. We find that the microcavity-induced optical confinement controls the efficiency and spectral selection of photocurrent generation in the integrated graphene device. A twenty-fold enhancement of photocurrent is demonstrated. The optical cavity also determines the spectral properties of the electrically excited thermal radiation of graphene. Most interestingly, we find that the cavity confinement modifies the electrical transport characteristics of the integrated graphene transistor. Our experimental approach opens up a route towards cavity-quantum electrodynamics on the nanometre scale with graphene as a current-carrying intra-cavity medium of atomic thickness. Graphene, an atomic monolayer formed by carbon hexagons, is a material with extraordinary electrical and optical properties [1] , [2] , [3] . Consequently, there is a growing interest in graphene optoelectronics [4] and first demonstrations of graphene-based photodetectors [5] , optical modulators [6] , plasmonic devices [7] , [8] and ultra-fast lasers [9] have been reported. Because of its two-dimensional geometry, graphene is ideally suited for enclosure within a planar λ /2 microcavity, a photonic structure that confines optical fields between two highly reflecting mirrors with a spacing of only one half wavelength of light. The optical confinement could provide a powerful means of controlling the otherwise featureless optical absorption [10] as well as the spectrally broad thermal emission [11] , [12] of graphene. The concept of optical confinement of graphene enables a new class of functional devices as, for example, spectrally selective and highly directional light emitters, detectors and modulators. Moreover, it opens up the opportunity for investigating fundamental, cavity-induced modifications of light–matter interaction in graphene. According to Fermi's golden rule [13] , the spontaneous photon emission (absorption) rate is determined by the local photonic mode density that can be significantly altered inside an optical microcavity [14] . The cavity-induced confinement enables the enhancement [15] or the inhibition [16] of the light emission (absorption) rate of the intra-cavity medium. The in-plane transition dipole moment of the intra-cavity medium couples to the longitudinal cavity mode of the cavity with wavelength-dependent efficiency, and the coupling strength is maximized at the antinode of the optical field located at the cavity centre [17] , [18] . 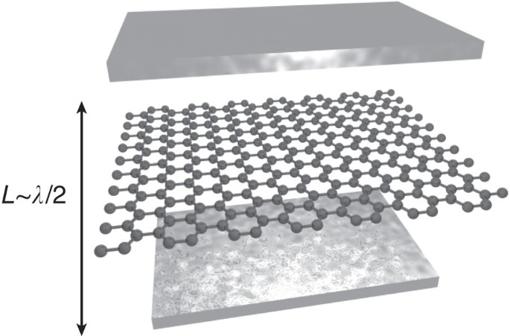Figure 1: Microcavity-induced optical confinement of graphene. Visualization of a graphene layer located at the centre of a planar opticalλ/2 microcavity. Optical fields with wavelengthλare confined in the direction perpendicular to the cavity mirrors with spacingL. The optical coupling is maximized if the graphene layer is oriented parallel to the cavity mirrors. Figure 1 visualizes the principle of confining graphene by a planar optical cavity. Figure 1: Microcavity-induced optical confinement of graphene. Visualization of a graphene layer located at the centre of a planar optical λ /2 microcavity. Optical fields with wavelength λ are confined in the direction perpendicular to the cavity mirrors with spacing L . The optical coupling is maximized if the graphene layer is oriented parallel to the cavity mirrors. Full size image The cavity-induced rate enhancement, or Purcell-effect, has already been demonstrated with quasi 2D quantum wells, as well as quasi 1D and 0D systems such as atoms, molecules, quantum dots and other nanoparticles [14] . However, embedding a truly 2D material such as graphene into a planar cavity has not been reported so far. Yet such an approach is highly desirable for two main reasons. First, the coupling area, that is, the spatial overlap between graphene and the cavity, can be extended to the micrometre scale within the two dimensions of the cavity plane, whereas preserving the optical confinement of graphene with respect to the cavity normal on the length scale of λ/ 2 (see Fig. 1 ). This is important because optical transitions in graphene are associated with in-plane transition dipole moments (π–π* transitions), thus rendering the 1D planar cavity confinement highly efficient. Second, the Fermi energy and density-of-states of graphene can be tuned easily by directly connecting it to electrodes, thus enabling charge carrier control, electrical transport and heating within the active area of the cavity. Graphene hence opens a unique experimental approach towards cavity-quantum electrodynamics on the nanometre scale with a current-carrying intra-cavity medium of atomic thickness. In this paper, we report the monolithic integration of a graphene transistor with a planar optical microcavity. We find that both photocurrent generation as well as electrically excited thermal light emission of graphene can be controlled by the spectral properties of the microcavity. The device constitutes a first implementation of a cavity-enhanced graphene light detector, as well as a demonstration of a fully integrated, narrow-band thermal light source. Most importantly, the optical confinement of graphene by the microcavity profoundly modifies the electrical transport characteristics of the integrated graphene transistor. 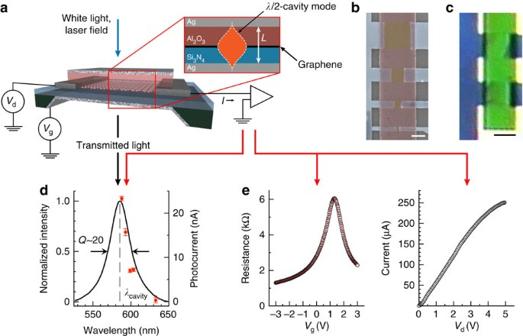Figure 2: Microcavity-controlled graphene transistor and photocurrent generation. (a) Schematic representation and electrical interconnection of the device. Inset: cross-sectional view of the device. The graphene sheet is embedded between two Ag mirrors and separated by two dielectric layers (Si3N4; Al2O3). The thicknessLof the dielectric stack between the cavity mirrors determines the resonance wavelengthλof the optical microcavity. Also shown is a visualization of the intensity profile of the fundamentalλ/2 cavity mode. (b) Top-view scanning electron microscope false colour image of the device; graphene sheets (yellow), Pd contacts (blue) Ag mirror (red). Scale bar, 2 μm. (c) Optical white light transmission micrograph of the device. The fundamental cavity mode is spectrally located atλcavity=585 nm, which appears green to the eye. Scale bar, 4 μm. (d) Optical transmission spectrum of the device (black line) measured with white light illumination reveals the cavity resonance atλcavity=585 nm having a cavity-Qof 20. The measured laser-induced photocurrent amplitude (red dots) samples the spectral profile of the optical cavity resonance. (e) Electrical transfer (left) and output (right) characteristics of the device; the fit (red solid line) to the transfer data (open symbols) is explained in the main text. Device design Figure 2a outlines our novel integration principle: an electrically contacted single layer of graphene is embedded between two optically transparent, dielectric thin films made of Si 3 N 4 and Al 2 O 3 , respectively. The dielectric layers are enclosed by two metallic (Ag, Au) mirrors with a spacing L that determines the resonance wavelength λ cavity of the microcavity (see Methods and ref. 18 ). A novel multi-step manufacturing process (see Methods ) allows us to define device area and cavity mirror spacing with nanometre precision and to build a series of devices that satisfy the specific requirements of different optoelectronic experiments. For photocurrent studies, we designed the cavity resonance to match the tuning range of the laser system at hand (~580 nm). For thermal emission studies, we designed the cavity resonance to be spectrally located within the detection range of the spectroscopic unit (~925 nm). In principle, all the measurements can be performed on the same device, whereas the efficiencies of light absorption and emission are largely determined by the optical properties of the cavity. Figure 2: Microcavity-controlled graphene transistor and photocurrent generation. ( a ) Schematic representation and electrical interconnection of the device. Inset: cross-sectional view of the device. The graphene sheet is embedded between two Ag mirrors and separated by two dielectric layers (Si 3 N 4 ; Al 2 O 3 ). The thickness L of the dielectric stack between the cavity mirrors determines the resonance wavelength λ of the optical microcavity. Also shown is a visualization of the intensity profile of the fundamental λ /2 cavity mode. ( b ) Top-view scanning electron microscope false colour image of the device; graphene sheets (yellow), Pd contacts (blue) Ag mirror (red). Scale bar, 2 μm. ( c ) Optical white light transmission micrograph of the device. The fundamental cavity mode is spectrally located at λ cavity =585 nm, which appears green to the eye. Scale bar, 4 μm. ( d ) Optical transmission spectrum of the device (black line) measured with white light illumination reveals the cavity resonance at λ cavity =585 nm having a cavity- Q of 20. The measured laser-induced photocurrent amplitude (red dots) samples the spectral profile of the optical cavity resonance. ( e ) Electrical transfer (left) and output (right) characteristics of the device; the fit (red solid line) to the transfer data (open symbols) is explained in the main text. Full size image Microcavity-controlled light detection Figure 2b–e reports the device characterization by electrical, optical and optoelectronic measurements: to characterize the electronic device properties, we measure both electrical transfer and output characteristics of the integrated graphene transistor ( Fig. 2e ). We apply a bias voltage along the graphene sheet and use one of the metallic cavity mirrors as a gate electrode ( Fig. 2a ). We fit the measured electrical transfer characteristics based on the model reported in ref. 19 and extract the device parameters that demonstrate the quality of the graphene sheet and the Pd-graphene contacts: we find a carrier mobility μ =2350 cm 2 V −1 s −1 , a residual carrier density n 0 =4.9×10 11 cm −2 , an electrical-resistance ratio R max / R min =5, and a specific contact resistance R c =0.265 kΩ μm. To characterize the optical properties of the device, we illuminate the cavity with white light from the top (see Fig. 2a ) and spectrally analyse the transmitted light. This way, we determine the resonance wavelength λ cavity and the cavity quality factor Q = λ cavity /Δ λ cavity , where Δ λ cavity is the spectral full-width-at-half-maximum (FWHM) of the peak at λ cavity in the measured transmission spectrum. In the present case ( Fig. 2d ), we obtain λ cavity =585 nm and cavity- Q =20. We employ photocurrent generation in graphene [20] to probe electronically the optical absorption of the graphene layer inside the device. We focus a laser beam on one of the microcavity mirrors, tune the laser wavelength across the optical resonance, and measure the photocurrent generated inside the biased graphene layer by means of a lock-in technique. The functional dependence of the photocurrent amplitude on laser wavelength ( Fig. 2d , red circles) matches the spectral profile of the cavity resonance as measured by white light transmission micro-spectroscopy ( Fig. 2d , solid line). By tuning the laser wavelength to λ laser =583 nm, on resonance with the microcavity, we obtain a photocurrent amplitude of 23.3 nA, while we measure only 1.2 nA for laser illumination at λ laser =633 nm. The photocurrent modulation by a factor of 20 demonstrates that the device acts as a light detector with spectral selectivity. In contrast, the photocurrent amplitude of a non-confined graphene transistor varies by less than a factor of two if we tune the laser excitation wavelength across the same spectral interval. Microcavity-controlled thermal light emission We now investigate the light-emission properties of non-confined graphene and compare it to the microcavity-controlled graphene transistor. By applying a bias voltage across the non-confined graphene device using source and drain electrodes ( Fig. 3a ), the electrical current heats up the graphene layer and thermal light emission sets in, as reported previously [11] , [12] . As shown in Fig. 3b , the electrically excited, thermal emission spectrum of graphene in free, non-confined space exhibits a featureless exponential tail that shifts from the near-infrared towards the visible spectral range as a function of injected electrical power. The temperature values are extracted by fitting the measured emission spectra based on a model of a two-dimensional black body (see Methods and ref. 21 ). 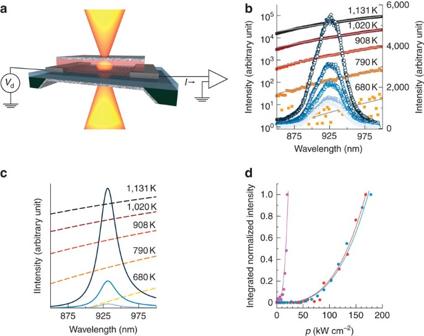Figure 3: Electrically excited microcavity-controlled graphene thermal emitter. (a) The schematic visualizes how thermal light emission is generated by applying a drain bias and how thermal radiation couples to the optical cavity mode. (b) Thermal near-infrared emission spectra measured for a cavity-confined (open circles) and a non-confined (filled squares) graphene transistor. The emission spectra of the cavity-controlled graphene transistor displays the optical resonance of the cavity atλcavity=925 nm. The lefty-axis is the intensity of the non-confined emission (log scale), whereas the righty-axis is the intensity of the confined emission (linear scale). The indicated temperatures are derived by fitting the non-confined thermal radiation spectra to Planck's law (seeMethods). (c) Simulated spectra of cavity-controlled thermal radiation (solid lines) and non-confined thermal radiation (dashed lines) modelled by assuming that the cavity resonance is spectrally located atλcavity=925 nm and has a spectral full width at half maximum of 30 nm. (d) Spectrally integrated light intensity as function of electrical power for three devices with different channel sizes (red 1×1 μm2, blue 2×2 μm2, purple 4×4 μm2). The solid lines areT3fits assuming that the dissipated electrical power is proportional to the temperatureTin the graphene sheet. Figure 3: Electrically excited microcavity-controlled graphene thermal emitter. ( a ) The schematic visualizes how thermal light emission is generated by applying a drain bias and how thermal radiation couples to the optical cavity mode. ( b ) Thermal near-infrared emission spectra measured for a cavity-confined (open circles) and a non-confined (filled squares) graphene transistor. The emission spectra of the cavity-controlled graphene transistor displays the optical resonance of the cavity at λ cavity =925 nm. The left y -axis is the intensity of the non-confined emission (log scale), whereas the right y -axis is the intensity of the confined emission (linear scale). The indicated temperatures are derived by fitting the non-confined thermal radiation spectra to Planck's law (see Methods ). ( c ) Simulated spectra of cavity-controlled thermal radiation (solid lines) and non-confined thermal radiation (dashed lines) modelled by assuming that the cavity resonance is spectrally located at λ cavity =925 nm and has a spectral full width at half maximum of 30 nm. ( d ) Spectrally integrated light intensity as function of electrical power for three devices with different channel sizes (red 1×1 μm 2 , blue 2×2 μm 2 , purple 4×4 μm 2 ). The solid lines are T 3 fits assuming that the dissipated electrical power is proportional to the temperature T in the graphene sheet. Full size image In contrast, the thermal emission spectrum of a microcavity-controlled graphene transistor displays a single, narrow peak at λ cavity =925 nm having a FWHM of 50 nm ( Fig. 3b ), providing a 140-fold spectral narrowing as compared with the simulated free-space thermal spectrum at T =650 K. It is important to note that this is not merely a spectral filtering effect, but that thermal radiation cannot be emitted by the graphene layer at all if the thermal radiation wavelength λ thermal is larger than λ cavity because of the optical confinement, or, in other words, the cavity-induced inhibition of spontaneous emission. This constitutes the first demonstration of a current-driven, microcavity-controlled thermal light source. The spectral peak position of the emission peak does not shift as a function of injected electrical power. The simulated emission spectra in Fig. 3c reproduce the overall shape of their experimental counterparts very well (for details, see Methods ). Further data analysis reveals that microcavity-controlled thermal radiation is emitted into a narrow lobe with a total angular width of 24° (FWHM) only (see Supplementary Methods and Supplementary Fig. S1 ). The integral over the microcavity-controlled light intensity is plotted as function of the injected electrical power in Fig. 3d for three different devices. The power dependences reveal that the integrated light intensity is proportional to T 3 as expected from the Stefan-Boltzmann law in two dimensions [21] . Here we assume that the electrical power density p T , which is validated by measurements in non-confined space (see Supplementary Fig. S2 ). We now establish the physical concept of cavity-controlled thermal light generation in graphene. The graphene layer initially heats up due to carrier scattering. The emission of long-wavelength thermal radiation at λ thermal > λ cavity is however inhibited by the cavity. As the temperature in the graphene sheet increases as a function of the electrical power density p , the thermal distribution inside the graphene layer spectrally shifts towards λ cavity ( Fig. 3b ) and, at a threshold temperature T cavity , eventually enables the emission of a significant fraction of photons at λ thermal λ cavity . We note that the temperature T cavity and the corresponding threshold power density p cavity depend on device parameters, that is, the carrier mobility μ , the channel area and λ cavity . For the device in Fig. 3b , we find T cavity ≈650 K and p cavity =90 kW cm −2 . Based on Wien's law in two dimensions, [21] we estimate that the graphene layer would have to be heated up to T cavity,optimum ≈ hc /3.92 k B λ cavity ≈4,000 K to maximize the light output at λ cavity =925 nm. In this case, the intensity maximum of the thermal-radiation distribution would overlap with the cavity resonance at λ cavity , resulting in a peak population of the cavity mode by thermal photons. Note that we designed microcavity devices specifically for performing the thermal emission spectroscopy in the near-infrared to take advantage of the favourable experimental conditions, that is, the high sensitivity and detection yield of the CCD array at hand. The optimum light-emitting performance, however, is expected to be in the mid-infrared spectral range. Assuming device operation at, for example, T cavity =650 K, we estimate a maximum thermal light output at λ thermal ≈5.6 μm. Future work should hence extend the spectral range towards the terahertz regime. Transport in microcavity-controlled graphene transistors Finally, we discuss modifications of electrical transport in optically confined graphene by correlating the electrical current and the spectrally integrated thermal radiation. In Fig. 4a–c , we show the electrical output characteristics of a graphene transistor in non-confined space. The electrical current in the graphene layer saturates in the high bias regime, whereas thermal light emission sets in as it shifts into the detection range. Performing the same experiment for a cavity-controlled graphene transistor with identical dimensions, we find that the electrical output characteristic is qualitatively different (see Fig. 4d–f ) and we can identify three different regimes by comparing electrical transport and light emission properties. In the sub-threshold regime (I), the electrical current saturates and the graphene layer heats up while the cavity-induced inhibition of spontaneous emission for λ thermal > λ cavity prevents off-resonant thermal radiation. In the threshold regime (II), the temperature of the graphene sheet has reached the critical value T cavity enabling light emission at λ thermal λ cavity . In the above-threshold regime (III), the initial electrical current saturation is lifted and the electrical resistance drops as function of electrical power density. 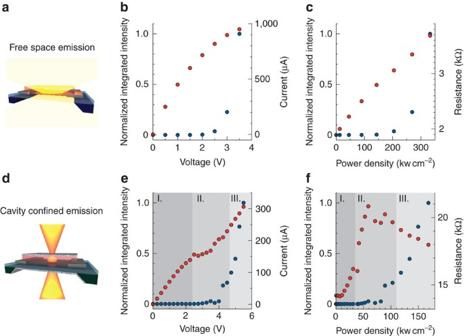Figure 4: Optical confinement and electrical transport in a microcavity-controlled graphene transistor. (a) Schematic illustration of the sample layout. (b) Normalized and integrated emitted light intensity (blue) and electrical current (red) as a function of bias voltage measured with a non-confined graphene transistor and (c) the integrated light intensity (blue) and the electrical resistance (red) plotted as a function of electrical power density. (d) Schematic illustration of the sample layout. (e) Normalized integrated emitted light intensity (blue) and electrical current (red) as a function of bias voltage measured with a microcavity-controlled graphene transistor and (f), the integrated light intensity (blue) and the electrical resistance (red) plotted as a function of electrical power density. Three regimes can be identified: (I) sub-threshold, (II) threshold and (III) above threshold, respectively. Figure 4: Optical confinement and electrical transport in a microcavity-controlled graphene transistor. ( a ) Schematic illustration of the sample layout. ( b ) Normalized and integrated emitted light intensity (blue) and electrical current (red) as a function of bias voltage measured with a non-confined graphene transistor and ( c ) the integrated light intensity (blue) and the electrical resistance (red) plotted as a function of electrical power density. ( d ) Schematic illustration of the sample layout. ( e ) Normalized integrated emitted light intensity (blue) and electrical current (red) as a function of bias voltage measured with a microcavity-controlled graphene transistor and ( f ), the integrated light intensity (blue) and the electrical resistance (red) plotted as a function of electrical power density. Three regimes can be identified: (I) sub-threshold, (II) threshold and (III) above threshold, respectively. Full size image We have observed electrical transport modifications similar to those shown in Fig. 4 in all functional graphene-cavity devices (a total of five), that is, those that allowed for thermal light generation (see Supplementary Fig. S3 ). In all cases, the saturation currents in regime I were lower than those obtained in the non-confined reference devices (same contacts and dielectric layers, no metal mirrors). One can rationalize this observation by assuming that the onset of current saturation in graphene depends on temperature and that the degree of self heating is determined by the thermal coupling of graphene to its local environment, captured by the thermal conductance r as suggested in ref. 22 . The saturation current j in the graphene layer would then be proportional to r . This implies that cavity-induced variations of r with respect to the non-confined reference value r 0 will lead to variations of the saturation current j and, accordingly, to the temperature in the graphene layer. In this scenario, the cavity-induced inhibition of the radiative thermal relaxation leads to enhanced self heating of the graphene layer and an onset of current saturation at lower electrical power levels as compared with the non-confined case. Based on the experimental transport data and the self-heating model presented in ref. 22 , we estimate temperature changes as high as Δ T =100 K when compared with the same graphene transistor in non-confined space (see Supplementary Methods and Supplementary Fig. S4 ). In this context, we point out that the amount of heat that is radiatively dissipated from the graphene sheet is very small, orders of magnitude smaller than the amount of energy that is dissipated non-radiatively [11] (see Supplementary Fig. S5 ). It is clear then that a proper model of electrical transport and its temperature dependence in a microcavity-controlled graphene transistor should account for the current-induced self-heating of graphene that is affected by both the non-radiative heat transfer through dielectric interfaces and metal contacts, and the microcavity-controlled, radiative heat transfer. In summary, we have demonstrated that a microcavity-controlled graphene transistor can act as a spectrally selective light detector and emitter with greatly enhanced sensitivity. Moreover, we have found that the cavity-induced optical confinement modifies graphene's electrical transport characteristics, an effect that may have important implications for nanoelectronics as well as cavity quantum electrodynamics. Note added in proof: A photodetection study of graphene inside a planar optical microcavity was reported while this work was under consideration (Furchi, M. et al . Microcavity-integrated graphene photodetector. Nano Lett. doi: 10.1021/nl204512x (2012)). Device fabrication Graphene sheets are produced via micromechanical cleavage of graphite on Si substrates covered with 300 nm of SiO 2 layer [23] . Single-layer graphene is identified by a combination of optical microscopy and Raman spectroscopy [24] , [25] . Three layers of 950 K poly(methyl methacrylate) (PMMA) are then spin coated on the substrates where flakes are deposited. The samples are subsequently immersed in de-ionized (DI) water at 90 °C for 2 h, resulting in the detachment of the polymer film, due to the intercalation of water at the polymer–SiO 2 interface. Graphene flakes stick to the PMMA film, and can thus be removed from the original substrate. The target substrate is a suspended Si 3 N 4 layer [n(Si 3 N 4 )≈2] with a thickness of 50 nm and an area of 50×50 μm 2 , supported by a Si frame having a thickness of 200 μm. We defined metallic markers by e-beam lithography and e-beam evaporation of 5 nm Ti and 50 nm Au on the target substrate. These markers are used for orientation during the transfer process and re-alignment for all following e-beam lithography steps. The PMMA+graphene film is transferred onto the suspended Si 3 N 4 layer. Because a thin layer of water is trapped at the substrate–polymer interface, the latter can be moved across the target substrate allowing accurate positioning of a chosen graphene flake onto a specific location on the Si 3 N 4 membrane. The sample is then left to dry, and finally PMMA is dissolved by acetone drop casting followed by immersion, resulting in the gentle release of the selected graphene flake on the target substrate. Success of the transfer is confirmed by Raman spectroscopy, which also proves the absence of process-induced structural defects. Metallic contacts are fabricated by e-beam lithography and sequential deposition of 0.5 nm Ti and 50 nm Pd by e-beam evaporation. In a next step, the selected single-layer graphene are shaped by oxygen plasma etching into different sizes (0.5×0.5 μm 2 , 1×1 μm 2 , 2×2 μm 2 and 4×4 μm 2 ). We then deposit a nucleation layer of 2 nm Al on top of the single-layer graphene to ensure homogeneous growth [26] , followed by an Al 2 O 3 layer (n(Al 2 O 3 )≈1.7) grown by atomic layer deposition of varying thickness. The chosen thicknesses of the intra-cavity dielectrics determine the resonance wavelength of the optical microcavity. To make the devices electrically accessible, we pattern openings over the large contact pads by e-beam lithography and etch away the Al 2 O 3 in 40% phosphoric acid by weight at a temperature of T =50 °C (etch rate ~10 nm/2 min) utilizing the PMMA resist as the etch mask. Cavity mirrors are prepared by depositing a 30 nm Ag (Au) globally on the backside of the sample by e-beam evaporation. An additional e-beam lithography step is necessary for the local definition of the top cavity mirror followed by deposition of 60 nm Ag (Au) to ensure devices can still be addressed electrically (see Supplementary Figs S6 and S7 ). Simulation of microcavity spectra Transmission and reflection spectra of the planar microcavity are simulated by using a transfer matrix method for multilayer stacks [27] . The stack used in the simulation consists of Ag(60 nm)/Al 2 O 3 (0–100 nm)/Si 3 N 4 (50 nm)/Ag(30 nm). The simulations reproduce well the experimental results obtained from a set of reference samples (see Supplementary Fig. S8 ). The thermal emission spectra of graphene in free, non-confined space are fitted with the spectral density model of the two-dimensional black-body radiation given in ref. 21 and the temperature is extracted for each electrical power density level. The microcavity-controlled thermal emission spectra of graphene are then simulated for the same temperatures by superimposing a single Lorentzian at λ cavity =925 nm with a FWHM of 30 nm on the spectral density of the two-dimensional black-body radiation discussed above. Note that, as compared with the measured white-light transmission spectrum of the same device, the peak in the thermal emission spectrum is blue shifted by 20 nm and broadened by a factor of 2 (see Supplementary Fig. S1 ). This is mainly due to the detection with high numerical aperture, NA=0.8, leading to wavelength-dependent variations of the collection efficiencies for on- and off-axis cavity emissions [18] , an effect that is not accounted for in the present model. How to cite this article: Engel, M. et al . Light-matter interaction in a microcavity-controlled graphene transistor. Nat. Commun. 3:906 doi: 10.1038/ncomms1911 (2012).